Activity of the mitochondrial calcium uniporter varies greatly between tissues The mitochondrial calcium uniporter is a highly selective channel responsible for mitochondrial Ca 2+ uptake. The mitochondrial calcium uniporter shapes cytosolic Ca 2+ signals, controls mitochondrial ATP production, and is involved in cell death. Here using direct patch-clamp recording from the inner mitochondrial membrane, we compare mitochondrial calcium uniporter activity in mouse heart, skeletal muscle, liver, kidney and brown fat. Surprisingly, heart mitochondria show a dramatically lower mitochondrial calcium uniporter current density than the other tissues studied. Similarly, in Drosophila flight muscle, mitochondrial calcium uniporter activity is barely detectable compared with that in other fly tissues. As mitochondria occupy up to 40% of the cell volume in highly metabolically active heart and flight muscle, low mitochondrial calcium uniporter activity is likely essential to avoid cytosolic Ca 2+ sink due to excessive mitochondrial Ca 2+ uptake. Simultaneously, low mitochondrial calcium uniporter activity may also prevent mitochondrial Ca 2+ overload in such active tissues exposed to frequent cytosolic Ca 2+ activity. Mitochondrial Ca 2+ uptake has long been recognized as instrumental in cellular physiological and pathophysiological conditions [1] , [2] , [3] . It controls the rate of mitochondrial ATP production [4] , [5] , shapes cytosolic Ca 2+ signals in heart and other tissues [6] , [7] , [8] , [9] , [10] , modulates the contraction-relaxation cycle of skeletal muscle [11] , [12] , regulates immunological synapses [13] , and is involved in cell death [1] , [14] , [15] . Cytosolic Ca 2+ influx into the mitochondrial matrix is mediated primarily by the mitochondrial calcium uniporter (MCU) [10] , [16] , [17] . Patch-clamp studies in vesicles of the native inner mitochondrial membrane (IMM, mitoplasts) have demonstrated that the MCU is a highly selective Ca 2+ channel with unique properties [18] . Functional characterization of the MCU has been followed by a search for molecular candidates, and to date two molecules, MICU1 and MCU, have been shown to be important for the MCU activity [19] , [20] , [21] , [22] . Mitochondrial Ca 2+ uptake has been primarily studied indirectly using ion flux assays in suspensions of isolated mitochondria and by calcium imaging in intact cells. These studies have led to the identification and characterization of the phenomenon of mitochondrial Ca 2+ uptake in vitro [17] , [23] and demonstrated that this uptake occurs under physiological conditions in intact cells despite the low transport affinity of MCU for Ca 2+ (refs 24 , 25 ). However, these methods do not measure MCU activity directly; thus, mitochondrial potential (ΔΨ m ), matrix pH, and ion gradients across the IMM cannot be accurately controlled [17] , [23] , [25] . Therefore, it is not clear whether mitochondrial Ca 2+ uptake mediated by the MCU is the same among different tissues and whether any differences can influence the physiology of these tissues. Scarce evidence for the tissue heterogeneity of Ca 2+ uptake mediated by the MCU exists [26] , and it is still generally assumed that the activity of the Ca 2+ conductance associated with the MCU is the same among different tissues [27] , [28] . Here we applied the patch-clamp technique to mitoplasts isolated from a variety of excitable, as well as non-excitable mouse tissues. This method allows for the comparison of MCU activity in different tissues under tightly controlled conditions of ΔΨ m , Ca 2+ and H + gradients across the IMM [18] . Unexpectedly, of all mouse tissues tested (heart, skeletal muscle, liver, kidney and brown fat), heart mitochondria manifested the lowest MCU activity. The MCU current density in heart mitochondria was 30 times smaller than that in skeletal muscle. The relevance of this evidence was further corroborated by our observation that mitochondria from the highly metabolically active Drosophila flight muscle manifests almost no MCU activity, at variance with other populations of Drosophila mitochondria, which indeed possess large current densities. Our results are the first direct evidence that the amount of Ca 2+ uptake mediated by the MCU varies between tissues. The low mitochondrial Ca 2+ conductance observed in tissues with a high mitochondrial volume density and that are continuously subjected to high cytosolic Ca 2+ elevations, such as mouse heart and Drosophila flight muscle, is likely to be essential in having normal intracellular Ca 2+ signaling, as well as protecting these active tissues from toxic mitochondrial Ca 2+ overload. Mitochondrial Ca 2+ current varies among mouse tissues The unique conductance that mediates Ca 2+ uptake into mitochondria was shown to be a very selective Ca 2+ channel with high current density in monkey-derived COS7 cells [18] . In that study, the patch-clamp technique applied to mitoplasts (obtained by hypotonic shock-disruption of the outer mitochondrial membrane (OMM) of isolated COS7 cell mitochondria) was used to record Ca 2+ currents carried by the MCU [18] . Yet, the success rate in formation of the ‘whole-mitoplast’ mode of the patch-clamp technique to record currents across the whole native IMM was low. French press employed to mechanically subfractionate mitochondria was advantageous over others methods, as mitoplasts with both structural and functional integrity were obtained [29] . Here we patch-clamped mitoplasts derived from French-pressed mitochondria of mouse heart, skeletal muscle, liver, kidney and brown adipose tissue. The French press protocol used to obtain vescicles of the IMM proved instrumental in increasing the yield of reliable and stable whole-mitoplast recordings from all tissues studied. 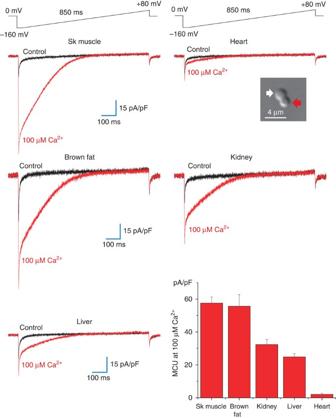Figure 1: Mitochondrial Ca2+conductance in different mouse tissues. Whole-mitoplast current recorded before (black traces) and after (red traces) application of 100 μM Ca2+to the bath solution. Currents were elicited by a voltage-ramp protocol (shown above) from different mouse tissues (as indicated). Note that brown fat mitoplasts were isolated from mice deficient for uncoupling protein 1 (UCP1, see methods). Whole-mitoplastIMCUwas normalized to the membrane capacitance (Cm) in all tissues examined. Picture in inset, representative transmitted differential interference contrast image of a mouse heart mitoplast obtained with French press. Note the figure 8-shaped form of the mitoplast. The lobe of the mitoplast containing only the IMM was less dense (white arrow) and clearly distinguishable from the lobe covered with the OMM (red arrow). Bottom right panel: Histogram showing averageIMCUcurrent densities in 100 μM Ca2+in different tissues. Current amplitudes were measured at 5 ms after stepping from 0 mV to −160 mV (see the voltage protocol). Note the lowIMCUcurrent density in heart compared with other tissues. Statistical data are represented as mean±s.e.m. Figure 1 (see picture in the inset) shows a differential interference contrast image of a mouse heart mitoplast obtained with the French press method. In 150 mM KCl solution, mitoplasts generated with the French press method normally have a figure 8-shaped form, as the IMM protrudes through one of small ruptures in the OMM to produce a bilobed vesicle. The lobe of the mitoplast covered with remnants of the OMM (inset, red arrow) appeared optically denser (as it contained two membranes) than the lobe consisting of the IMM only (inset, white arrow). After strorage on ice for several hours, mitoplasts assumed a round shape with the remnants of the OMM attached from one side (the so-called ‘cap’ region). We found that the newly prepared figure 8-shaped mitoplasts were the best choice for the formation of the whole-mitoplast mode, while the success rate in the formation of this mode with older round-shaped mitoplasts was lower. Figure 1: Mitochondrial Ca 2+ conductance in different mouse tissues. Whole-mitoplast current recorded before (black traces) and after (red traces) application of 100 μM Ca 2+ to the bath solution. Currents were elicited by a voltage-ramp protocol (shown above) from different mouse tissues (as indicated). Note that brown fat mitoplasts were isolated from mice deficient for uncoupling protein 1 (UCP1, see methods). Whole-mitoplast I MCU was normalized to the membrane capacitance ( C m ) in all tissues examined. Picture in inset, representative transmitted differential interference contrast image of a mouse heart mitoplast obtained with French press. Note the figure 8-shaped form of the mitoplast. The lobe of the mitoplast containing only the IMM was less dense (white arrow) and clearly distinguishable from the lobe covered with the OMM (red arrow). Bottom right panel: Histogram showing average I MCU current densities in 100 μM Ca 2+ in different tissues. Current amplitudes were measured at 5 ms after stepping from 0 mV to −160 mV (see the voltage protocol). Note the low I MCU current density in heart compared with other tissues. Statistical data are represented as mean±s.e.m. Full size image In the whole-mitoplast configuration, the addition of 100 μM Ca 2+ to the bath (the cytosolic face of the IMM) induced an inwardly rectifying Ca 2+ current, presumably carried by the MCU ( I MCU ). I MCU current density greatly varied among different tissues examined ( Fig. 1 ). I MCU current densities measured upon stepping from 0 mV to −160 mV were as follows: skeletal muscle, 58±4 pA/pF, n =10; brown adipose tissue, 56±7 pA/pF, n =6; kidney, 32±3 pA/pF, n =10; liver, 25±2 pA/pF, n =10; and heart, 2.1±0.6 pA/pF, n =8 ( Fig. 1 , histogram in the lower right panel, mean±s.e.). Surprisingly, I MCU in heart mitoplasts was the lowest among all tissues and as much as 30 times smaller than that in closely related skeletal muscle. In contrast, another hallmark conductance of the IMM, the inner membrane anion channel [30] , [31] , [32] , was present in all tissues examined (not shown) and showed no difference in activity between heart and skeletal muscle ( Fig. 2 ). 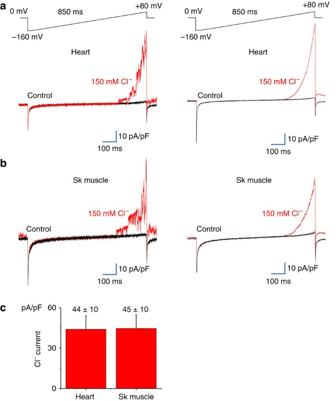Figure 2: Cl−current of the IMM of heart and skeletal muscle. (a) Left panel: representative whole-mitoplast current recorded from a mouse heart mitoplast before (black traces) and after (red traces) application of 150 mM Cl−to the bath solution. Pipette solution contained 4 mM Cl−. Currents were elicited by a voltage-ramp protocol (shown above). The whole-mitoplast Cl−current was normalized to the membrane capacitance (Cm). Right panel: Same experiment as in (a), but the traces represent an average of 30–50 original current traces to smooth out fluctuations of the outward Cl- current mediated by the large-conductance inner membrane anion channel (b) Left panel: representative whole-mitoplast current recorded from a mouse skeletal muscle mitoplast before (black traces) and after (red traces) application of 150 mM Cl-to the bath solution. Pipette solution contained 4 mM Cl−. Currents were elicited by a voltage-ramp protocol (shown above). The whole-mitoplast Cl−current was normalized to the membrane capacitance (Cm). Right panel: Same experiment as in (a), but the traces represent an average of 30–50 original current traces to smooth out fluctuations of the outward Cl- current mediated by the large-conductance anion channel. (c) Histogram comparing average Cl−current densities in 150 mM Cl−in mouse heart (n=4) and skeletal muscle (n=3). Current amplitudes were measured at +80 mV (see the voltage protocol) and normalized to theCm. Statistical data are represented as mean±s.e.m. Sk muscle, skeletal muscle. Figure 2: Cl − current of the IMM of heart and skeletal muscle. ( a ) Left panel: representative whole-mitoplast current recorded from a mouse heart mitoplast before (black traces) and after (red traces) application of 150 mM Cl − to the bath solution. Pipette solution contained 4 mM Cl − . Currents were elicited by a voltage-ramp protocol (shown above). The whole-mitoplast Cl − current was normalized to the membrane capacitance ( C m ). Right panel: Same experiment as in (a), but the traces represent an average of 30–50 original current traces to smooth out fluctuations of the outward Cl- current mediated by the large-conductance inner membrane anion channel ( b ) Left panel: representative whole-mitoplast current recorded from a mouse skeletal muscle mitoplast before (black traces) and after (red traces) application of 150 mM Cl - to the bath solution. Pipette solution contained 4 mM Cl − . Currents were elicited by a voltage-ramp protocol (shown above). The whole-mitoplast Cl − current was normalized to the membrane capacitance ( C m ). Right panel: Same experiment as in (a), but the traces represent an average of 30–50 original current traces to smooth out fluctuations of the outward Cl- current mediated by the large-conductance anion channel. ( c ) Histogram comparing average Cl − current densities in 150 mM Cl − in mouse heart ( n =4) and skeletal muscle ( n =3). Current amplitudes were measured at +80 mV (see the voltage protocol) and normalized to the C m . Statistical data are represented as mean±s.e.m. Sk muscle, skeletal muscle. Full size image As skeletal muscle and heart are related tissues and showed the higest and lowest I MCU current densities, respectively, we compared the biophysical properies of I MCU in these tissues to confirm that I MCU has the same properties in heart and skeletal muscle and is thus mediated by the same channel. I MCU shares the same properties in heart and skeletal muscle In both heart and skeletal muscle, I MCU elicited by voltage steps was primarily time-independent ( Fig. 3a ) and apparently lacked Ca 2+ -dependent inactivation, similar to what was previously reported for I MCU in COS7 cell mitochondria. As expected, in both tissues, I MCU was completely blocked by 50 nM RuR, a potent blocker of the MCU [17] , [18] ( Fig. 3b ). 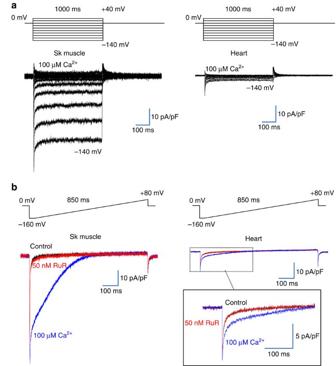Figure 3:IMCUis time-independent and blocked by RuR in skeletal muscle and heart. (a)IMCUelicited by a voltage-step protocol (as indicated on top, ΔV=20 mV) in skeletal muscle (left panel) and heart (right panel). (b)IMCUrecorded in the presence of 100 μM Ca2+(blue trace) was completely inhibited by 50 nM RuR (red trace) both in skeletal muscle (left panel) and heart (right panel). The black traces indicate the baseline recorded in the absence of Ca2+in the bath. Currents were normalized to the membrane capacitance to compareIMCUin heart and skeletal muscle. Voltage-ramp protocol is indicated on top. Sk muscle, skeletal muscle. Figure 3: I MCU is time-independent and blocked by RuR in skeletal muscle and heart. ( a ) I MCU elicited by a voltage-step protocol (as indicated on top, ΔV=20 mV) in skeletal muscle (left panel) and heart (right panel). ( b ) I MCU recorded in the presence of 100 μM Ca 2+ (blue trace) was completely inhibited by 50 nM RuR (red trace) both in skeletal muscle (left panel) and heart (right panel). The black traces indicate the baseline recorded in the absence of Ca 2+ in the bath. Currents were normalized to the membrane capacitance to compare I MCU in heart and skeletal muscle. Voltage-ramp protocol is indicated on top. Sk muscle, skeletal muscle. Full size image As expected for the Ca 2+ current, I MCU gradually increased as Ca 2+ concentrations in the bath were gradually elevated from 50 μM to 1 mM in both heart and skeletal muscle ( Fig. 4a ). Mg 2+ did not induce any I MCU ( Fig. 4b ), and the current traces in the presence of Mg 2+ in the bath solution were identical to the baseline (obtained in 200 nM RuR, data not shown). The addition of Ba 2+ to the bath induced I MCU , but the Ba 2+ current was much smaller than that induced by Ca 2+ ( Fig. 4b ). The permeability sequence for I MCU , Ca 2+ »Ba 2+ >Mg 2+ , ( Fig. 4c ) was the same as reported for the MCU studied by indirect methods [17] , [33] , [34] and by patch-clamping mitoplasts from COS7 cells [18] . Notably, the I MCU permeability sequence is unique, as most Ca 2+ channels conduct Ba 2+ better than Ca 2+ (ref. 35 ). 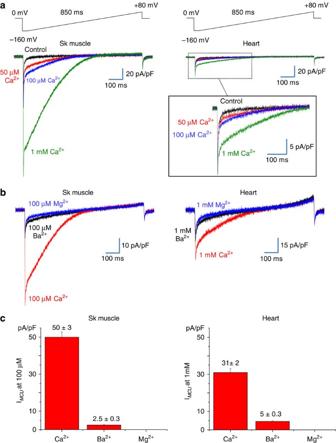Figure 4: Divalent cation permeability ofIMCUin skeletal muscle and heart. (a) RepresentativeIMCUrecorded in the presence of different concentrations of Ca2+in the bath: nominal Ca2+-free (black), 50 μM (red), 100 μM (blue), and 1 mM (green). Voltage-ramp protocol is indicated on top. (b) Left panel, RepresentativeIMCUrecorded from a skeletal muscle mitoplast in the presence of 100 μM Ca2+(red trace), Ba2+(black trace), and Mg2+(blue trace). Right panel, RepresentativeIMCUrecorded from a heart mitoplast in the presence of 1 mM Ca2+(red trace), Ba2+(black trace), and Mg2+(blue trace). (c) Histograms of the relative permeability ofIMCUto Ca2+, Ba2+and Mg2+in skeletal muscle (n=4, left panel) and heart (n=4, right panel). Current amplitudes were measured at 5 ms after stepping from 0 to −160 mV (see the voltage protocol in b). Statistical data are represented as mean±s.e.m. Sk muscle, skeletal muscle. Figure 4: Divalent cation permeability of I MCU in skeletal muscle and heart. ( a ) Representative I MCU recorded in the presence of different concentrations of Ca 2+ in the bath: nominal Ca 2+ -free (black), 50 μM (red), 100 μM (blue), and 1 mM (green). Voltage-ramp protocol is indicated on top. ( b ) Left panel, Representative I MCU recorded from a skeletal muscle mitoplast in the presence of 100 μM Ca 2+ (red trace), Ba 2+ (black trace), and Mg 2+ (blue trace). Right panel, Representative I MCU recorded from a heart mitoplast in the presence of 1 mM Ca 2+ (red trace), Ba 2+ (black trace), and Mg 2+ (blue trace). ( c ) Histograms of the relative permeability of I MCU to Ca 2+ , Ba 2+ and Mg 2+ in skeletal muscle ( n =4, left panel) and heart ( n =4, right panel). Current amplitudes were measured at 5 ms after stepping from 0 to −160 mV (see the voltage protocol in b). Statistical data are represented as mean±s.e.m. Sk muscle, skeletal muscle. Full size image Ca 2+ channels are selective for Ca 2+ due to the presence of high-affinity binding sites for Ca 2+ in the pore region [35] . Yet, under divalent-free (DVF) conditions, monovalent ions, which have significantly lower affinity for these binding sites, can still bind within the pore and permeate the Ca 2+ channels [35] . The monovalent current is inhibited when Ca 2+ is re-added to the bath solution, as Ca 2+ occupies the binding site in the pore and thus prevents monovalent ions from permeation. For plasma membrane Ca 2+ channels, the inhibition of the monovalent current by Ca 2+ occurs in the low micromolar range, whereas for the MCU of COS7 cells, this inhibition occurs in the low nanomolar range [18] . This finding identifies the MCU as the Ca 2+ channel with the highest known Ca 2+ selectivity. We, therefore, asked whether the MCU in mouse heart and skeletal muscle has the same high selectivity for Ca 2+ over monovalent ions as the MCU in COS7 cells. Under DVF conditions when bath and pipette solutions contained 110 mM Na + , we observed a quasi-linear current in both skeletal muscle and heart ( Fig. 5a–c , left panels for skeletal muscle and right panels for heart throughout). This Na + current was almost completely blocked by as low as 11 nM bath-free Ca 2+ , and 160 nM Ca 2+ totally abolished it ( Fig. 5a ). The Ca 2+ -sensitive Na + current was evidently mediated by the MCU that lost its selectivity under DVF conditions [18] , which was further confirmed by the fact that the Na + current was completely inhibited by 200 nM RuR ( Fig. 5b ). Similar to COS7 cell mitoplasts [18] , substitution of Na + for K + in the bath solution resulted in significantly lower monovalent current through the MCU, showing that the MCU was relatively impermeant to K + ions, in both skeletal muscle and heart ( Fig. 5c ). 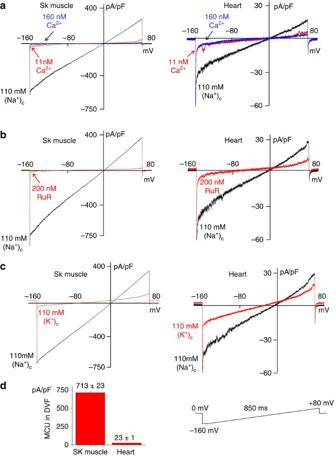Figure 5:IMCUis carried by Na+under DVF conditions in skeletal muscle and heart. (a) Na+current through the MCU under DVF conditions (black trace), and in the presence of either 11 nM (red trace) or 160 nM (blue trace) free Ca2+in the bath solution. Skeletal muscle (left panel), heart (right panel). Currents were normalized to membrane capacitance. The voltage protocol is shown in bottom of the figure. (b) The Na+current through the MCU before (black trace) and after (red trace) the addition of 200 nM RuR to the bath solution. (c) Monovalent current through the MCU in symmetrical 110 mM Na+(black trace) and after replacement of bath Na+with K+(red trace). (d) Histogram showing average densities of Na+current through the MCU in skeletal muscle (n=5) and heart (n=5). Current amplitudes were measured at 5 ms after stepping the membrane from 0 to −160 mV (see the voltage protocol). Statistical data are represented as mean±s.e.m. Sk muscle, skeletal muscle. Figure 5: I MCU is carried by Na + under DVF conditions in skeletal muscle and heart. ( a ) Na + current through the MCU under DVF conditions (black trace), and in the presence of either 11 nM (red trace) or 160 nM (blue trace) free Ca 2+ in the bath solution. Skeletal muscle (left panel), heart (right panel). Currents were normalized to membrane capacitance. The voltage protocol is shown in bottom of the figure. ( b ) The Na + current through the MCU before (black trace) and after (red trace) the addition of 200 nM RuR to the bath solution. ( c ) Monovalent current through the MCU in symmetrical 110 mM Na + (black trace) and after replacement of bath Na + with K + (red trace). ( d ) Histogram showing average densities of Na + current through the MCU in skeletal muscle ( n =5) and heart ( n =5). Current amplitudes were measured at 5 ms after stepping the membrane from 0 to −160 mV (see the voltage protocol). Statistical data are represented as mean±s.e.m. Sk muscle, skeletal muscle. Full size image The amplitude of the Na + current through the MCU was dramatically lower in heart (23±1 pA/pF, n =5) compared with skeletal muscle (713±23 pA/pF, n =5), which correlates well with the difference in amplitude of the Ca 2+ currents between these two tissues ( Fig. 5d ). We conclude that I MCU shares the same biophysical properties in heart and skeletal muscle, and these properties coincide with those of I MCU in COS7 cells [18] . Thus I MCU in heart and skeletal muscle is likely mediated by the same molecule, but heart mitochondria are endowed with dramatically lower MCU activity. I MCU is significantly larger in neonatal versus adult heart An important unresolved problem in cardiac Ca 2+ signalling is whether beat-to-beat elevations of mitochondrial [Ca 2+ ] occur in intact cardiomyocytes. Although this issue was addressed by several laboratories, a general consensus has not been reached. In a recent review, it has been noted that beat-to-beat oscillations might be developmentally regulated and occur in neonatal but not adult cardiomyocytes [7] . Although it has never been previously suggested, one of the specific reasons for this may be a higher Ca 2+ conductance of the IMM in neonatal cardiomyocytes as compared with adult cells. To test this hypothesis, we compared I MCU current density in cardiac mitoplasts isolated from newborn (2-day-old) and adult (>3 weeks) mice. Whole-mitoplast Ca 2+ currents from 2-day-old heart were recorded using the same solutions and voltage protocols used for adult heart. Interestingly, I MCU current density in neonatal mitoplasts measured with 100 μM Ca 2+ in the bath was five times larger (10.2±0.3 pA/pF) than in adult mitoplasts (2.1±0.5 pA/pF, see Fig. 6 ). These results demonstrate that the IMM of the neonatal heart has significantly larger Ca 2+ conductance as compared with adult heart, which may explain the age-related differences in beat-to-beat mitochondrial Ca 2+ accumulation in cardiomyocytes. 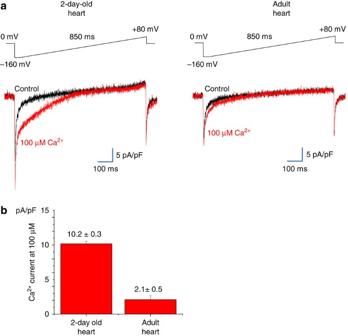Figure 6:IMCUcurrent density is significantly larger in neonatal compared with adult heart. (a) Left panel, RepresentativeIMCUelicited in the presence of 100 μM Ca2+(red traces) in a cardiac mitoplast isolated from a 2-day-old mouse. The black trace indicates the baseline recorded in the absence of Ca2+in the bath. Right panel, the same experiment performed with a cardiac mitoplast isolated from a 4-week-old (adult) mouse. Currents were elicited by a voltage-ramp protocol shown above. Whole-mitoplastIMCUwas normalized to theCm. (b) Histogram comparing averageIMCUcurrent densities in 2-day-old (n=5) and adult heart (n=8). Current amplitudes were measured at 5 ms after stepping from 0 to −160 mV (see the voltage protocol) and normalized to theCm. Statistical data are represented as mean±s.e.m. Figure 6: I MCU current density is significantly larger in neonatal compared with adult heart. ( a ) Left panel, Representative I MCU elicited in the presence of 100 μM Ca 2+ (red traces) in a cardiac mitoplast isolated from a 2-day-old mouse. The black trace indicates the baseline recorded in the absence of Ca 2+ in the bath. Right panel, the same experiment performed with a cardiac mitoplast isolated from a 4-week-old (adult) mouse. Currents were elicited by a voltage-ramp protocol shown above. Whole-mitoplast I MCU was normalized to the C m . ( b ) Histogram comparing average I MCU current densities in 2-day-old ( n =5) and adult heart ( n =8). Current amplitudes were measured at 5 ms after stepping from 0 to −160 mV (see the voltage protocol) and normalized to the C m . Statistical data are represented as mean±s.e.m. Full size image Tissue heterogeneity of I MCU in Drosophila Similar to our findings in mouse tissues, we found a dramatic difference in the density of the mitochondrial Ca 2+ current among Drosophila tissues. We first studied Ca 2+ currents in mitoplasts isolated from Drosophila flight muscle, which is of particular interest because this organ contracts at high frequencies. We obtained mitoplasts from thoraces of a Drosophila line in which the targeted mitochondrial expression of green fluorescent protein (GFP) in muscles was driven by crossing a upstream activating sequence-MitoGFP line with a muscle specific Mef2-Gal4 line (see Methods for details). Flight muscle mitochondria from this line express GFP in the matrix; hence, mitoplasts originating from it fluoresce. Drosophila thoraces were cleaned of legs to reduce contamination from leg muscle mitochondria. 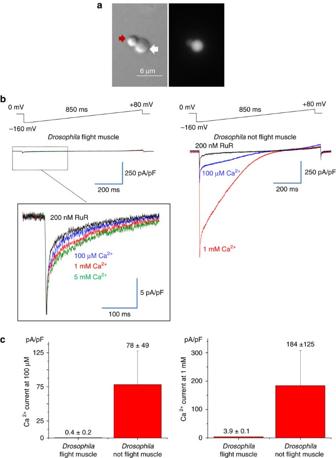Figure 7: Mitochondrial Ca2+conductance inDrosophilaflight muscle. (a) Representative transmitted left) and fluorescent (right) image of a French press-derived mitoplast isolated from flies expressing GFP targeted to the mitochondrial matrix of the flight muscle (Mef2 >MitoGFP). Note the figure 8-shaped form of the mitoplast. The lobe of the mitoplast containing only the IMM is less dense (white arrow) and clearly distinguishable from the lobe covered with the OMM (red arrow; compare withFig. 1inset). (b) Left panel: Representative mitochondrial Ca2+current recorded from aDrosophilaflight muscle mitoplast in different concentrations of bath Ca2+: 5 mM (green), 1 mM (red) and 100 μM (blue), and 5 mM Ca2+plus 200 nM RuR (black). Voltage-ramp protocol is indicated on top. Right panel: Representative mitochondrial Ca2+current recorded from aDrosophilanot flight muscle mitoplast in the presence of different concentrations of Ca2+in the bath: 1 mM (red) and 100 μM (blue), and 1 mM Ca2+plus 200 nM RuR (black). (c) Left panel: Histogram comparing average densities ofDrosophilamitochondrial Ca2+current at 100 μM in flight muscle (n=8) and not flight muscle tissues (n=3). Right panel: Histogram comparing average densities ofDrosophilamitochondrial Ca2+current at 1 mM in flight muscle (n=21) and not flight muscle tissues (n=6). Current amplitudes were measured at 5 ms after stepping the membrane from 0 to −160 mV (see the voltage protocol). Statistical data are represented as mean±s.e.m. Figure 7a shows a typical flight muscle GFP-fluorescent mitoplast used for patch-clamp recordings. Similar to mouse mitoplasts, Drosophila mitoplasts were obtained using the French press procedure and normally showed the same figure 8-shaped morphology (compare Figs 7a and 1 inset). The lobe that contained only the IMM was distinguishable from the optically denser lobe that was covered with the OMM and contained two membranes ( Fig. 7a , white and red arrows, respectively). Figure 7: Mitochondrial Ca 2+ conductance in Drosophila flight muscle. ( a ) Representative transmitted left) and fluorescent (right) image of a French press-derived mitoplast isolated from flies expressing GFP targeted to the mitochondrial matrix of the flight muscle (Mef2 >MitoGFP). Note the figure 8-shaped form of the mitoplast. The lobe of the mitoplast containing only the IMM is less dense (white arrow) and clearly distinguishable from the lobe covered with the OMM (red arrow; compare with Fig. 1 inset). ( b ) Left panel: Representative mitochondrial Ca 2+ current recorded from a Drosophila flight muscle mitoplast in different concentrations of bath Ca 2+ : 5 mM (green), 1 mM (red) and 100 μM (blue), and 5 mM Ca 2+ plus 200 nM RuR (black). Voltage-ramp protocol is indicated on top. Right panel: Representative mitochondrial Ca 2+ current recorded from a Drosophila not flight muscle mitoplast in the presence of different concentrations of Ca 2+ in the bath: 1 mM (red) and 100 μM (blue), and 1 mM Ca 2+ plus 200 nM RuR (black). ( c ) Left panel: Histogram comparing average densities of Drosophila mitochondrial Ca 2+ current at 100 μM in flight muscle ( n =8) and not flight muscle tissues ( n =3). Right panel: Histogram comparing average densities of Drosophila mitochondrial Ca 2+ current at 1 mM in flight muscle ( n =21) and not flight muscle tissues ( n =6). Current amplitudes were measured at 5 ms after stepping the membrane from 0 to −160 mV (see the voltage protocol). Statistical data are represented as mean±s.e.m. Full size image Drosophila flight muscle whole-mitoplast Ca 2+ currents were recorded using the same solutions and voltage protocols used for mouse mitoplasts. Interestingly, the Ca 2+ current induced by the gradual elevation of Ca 2+ in the bath from 100 μM to 5 mM was barely detectable ( Fig. 7b , left panel). Similar to the MCU current observed in mammalian mitoplasts, this small Ca 2+ current was RuR sensitive ( Fig. 7b , left panel). In contrast, when we specifically selected non-GFP mitoplasts that originated from tissues other than flight muscle of the Mef2 >MitoGFP flies, we were able to record robust whole-mitoplast RuR-sensitive Ca 2+ currents. Figure 7b shows a representative Ca 2+ current recorded from one such mitoplast. Interestingly, the density of the Ca 2+ current recorded from this particular mitoplast at 100 μM Ca 2+ (175 pA/pF) was significantly higher than that in any other mouse tissue examined ( Fig. 1 ). Overall, we recorded 31 Drosophila mitoplasts. Those mitoplasts originating from the flight muscle ( n =21) consistently showed a very-low Ca 2+ current both in 100 μM Ca 2+ (0.4±0.2 pA/pF, n =8) and in 1 mM Ca 2+ (3.9±0.1 pA/pF, n =13). Among the 10 mitoplasts derived from tissues other than flight muscle, six showed a Ca 2+ current significantly higher than that observed in flight muscle and four showed a very small Ca 2+ current. The six Drosophila mitoplasts with high Ca 2+ currents had very different values for current density (from 15 to 175 pA/pF in 100 μM Ca 2+ and from 11 to 800 pA/pF in 1 mM Ca 2+ ). The densities of the mitochondrial Ca 2+ currents from Drosophila flight muscle and other tissues are compared in Fig. 7c . In spite of the fact that the amplitude of the Ca 2+ current was extremely low in flight muscle mitoplasts, these mitoplasts had very large Cl − current ( Fig. 8 ) with the mean current density of 161±6 pA/pF at +80 mV, n =4. This is the first observation of the existence of a mitochondrial Cl − conductance in Drosophila . 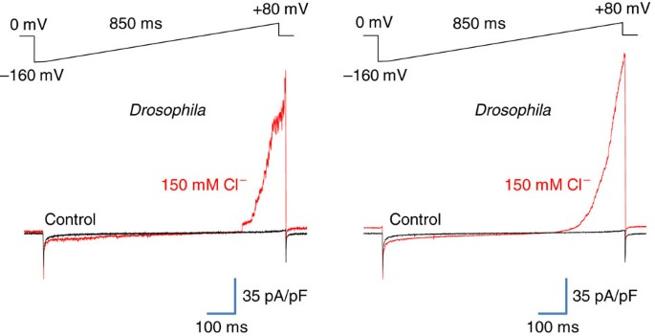Figure 8: Cl−current of the IMM ofDrosophilaflight muscle. Left panel: representative whole-mitoplast current recorded fromDrosophilaflight muscle before (black traces) and after (red traces) application of 150 mM Cl−to the bath solution. Pipette solution contained 2 mM Cl−. Currents were elicited by a voltage-ramp protocol (shown above). The whole-mitoplast Cl−current was normalized to the membrane capacitance (Cm). Right panel: Same experiment as in left panel, but the traces represent an average of 10–20 original current traces to smooth out fluctuations of the outward Cl−current mediated by a large-conductance channel. Figure 8: Cl − current of the IMM of Drosophila flight muscle. Left panel: representative whole-mitoplast current recorded from Drosophila flight muscle before (black traces) and after (red traces) application of 150 mM Cl − to the bath solution. Pipette solution contained 2 mM Cl − . Currents were elicited by a voltage-ramp protocol (shown above). The whole-mitoplast Cl − current was normalized to the membrane capacitance ( C m ). Right panel: Same experiment as in left panel, but the traces represent an average of 10–20 original current traces to smooth out fluctuations of the outward Cl − current mediated by a large-conductance channel. Full size image Therefore, as seen for mouse tissues, Drosophila tissues display significant differences in the mitochondrial Ca 2+ current density. RuR-sensitive Ca 2+ uptake into mitochondria isolated from the Drosophila -derived S2 cell line has recently been demonsrated [36] . This uptake and the RuR-sensitive Ca 2+ currents recorded from Drosophila mitoplasts are both likely to be mediated by a Drosophila homologue of the mammalian MCU. The phenomenon of MCU-mediated Ca 2+ uptake is one of the most interesting aspects of mitochondrial physiology. From its original discovery in the early 1960s (refs 37 , 38 ), this process was studied primarily with biochemical (ion flux studies) and optical (fluorescent proteins and indicators) methods, in either suspensions of isolated mitochondria or intact cells [3] , [17] , [23] , [25] . Although these methods identified the phenomenon of mitochondrial Ca 2+ uptake and provided its initial characterization, they did not allow for the reliable control of experimental conditions, and there have been significant variations in the rate of mitochondrial uptake measured in the same tissues by different labs [17] , [23] , [25] . Reliable comparisons of mitochondrial Ca 2+ uptake between different tissues have been difficult, and rare reports on the tissue-specific differences in MCU activity [26] have also been largely overlooked. Therefore, it was eventually concluded that mammalian mitochondria have a high rate of Ca 2+ uptake, and the MCU was described as a ‘high-capacity’ Ca 2+ transport mechanism [17] , [23] . Indeed, in many tissues, mitochondrial Ca 2+ uptake potently affects cytosolic Ca 2+ transients and causes a significant elevation of Ca 2+ in the mitochondrial matrix [10] , [24] . Thus, the present consensus in the field is that all mammalian mitochondria are endowed with approximately the same MCU activity and the same high ability to accumulate Ca 2+ . The demonstration that whole-IMM and unitary MCU currents can be recorded with the patch-clamp technique [18] overcame the technical limitations of the biochemical and optical methods. For the first time, this allowed direct studies of MCU activity under highly controlled conditions, such as exact potential across the IMM and exact concentrations for all ions on both sides of the IMM. Importantly, the patch-clamp technique allows for the dissection of single mechanisms involved in mitochondrial Ca 2+ transport and allows the characterization of MCU activity at the single organelle level. Here we applied the patch-clamp technique to compare the properties of Ca 2+ currents carried by the MCU in different mouse tissues. This study unexpectedly showed that the density of the MCU current in mouse heart is significantly lower than that in other mouse tissues. Interestingly, the MCU current density in heart was 30 times lower than that in closely related skeletal muscle. This dramatic difference is no likely the result of differences in the molecules responsible for mitochondrial Ca 2+ uptake in heart and skeletal muscle, as key biophysical properties of the mitochondrial Ca 2+ current in heart and skeletal muscle were the same and correlated well with the biophysical properties of the MCU in COS7 cells [18] . The very low density of the MCU current in heart was an unexpected finding, as accumulation of Ca 2+ into mitochondria in intact cardiac muscle has been previously demonstrated [6] , [7] , [8] , [39] , and mitochondrial Ca 2+ uptake in metabolically active tissues such as heart is perceived as important for the stimulation of mitochondrial ATP production and matching its rate with cytosolic Ca 2+ activity [7] , [8] , [10] . The paradoxically low MCU activity in heart, however, can be explained if we consider that mitochondria occupy up to 37% of the total cell volume in heart [40] . If these many heart mitochondria possessed a high ability to accumulate Ca 2+ , they could abolish the cytosolic Ca 2+ signalling necessary for heart contractile activity. Furthermore, because heart is characterized by frequent elevations of cytosolic Ca 2+ , robust mitochondrial Ca 2+ uptake would lead to extensive futile cycling of Ca 2+ across the IMM, resulting in low metabolic efficiency. Finally, the frequent elevation of cytosolic Ca 2+ could lead to mitochondrial Ca 2+ overload and dysfunction. Therefore, in heart, with its abundant mitochondria and frequent elevations in cytosolic Ca 2+ , it may be essential to limit MCU activity to preserve both a normal Ca 2+ -dependent heartbeat and mitochondrial integrity. In contrast, because skeletal muscle mitochondria occupy only about 5% of the cell volume [41] , [42] and are not exposed to frequent Ca 2+ elevations, limiting MCU activity in this tissue might not be necessary. It must be noted that although singular heart mitochondria have a limited ability to uptake Ca 2+ , their abundance can result in combined Ca 2+ accumulation comparable to other tissues. Interestingly, the density of the MCU current in cardiac mitoplasts isolated from newborn mice was about five times larger than that of adult mice. This demonstrates that the MCU activity can vary significantly not only between tissues but also during development. Important morphological changes occur during the first week after birth in cardiac myocytes, and the SR and mitochondrial networks are extensively remodeled [7] . In particular, mitochondrial volume density increases from about 20% in newborn to about 40% adults [43] , [44] . The age-related differences in the Ca 2+ conductance of the cardiac IMM reported here, together with the morphological changes in SR and mitochondrial network, may explain why beat-to-beat oscillations of mitochondrial Ca 2+ are usually observed in newborn and less often in adult cardiomyocytes [7] , [8] . Drosophila flight muscle is characterized by even higher Ca 2+ -dependent contractile activity than mouse heart, and mitochondria in this tissue occupy about 40% of the cell volume [45] , [46] . Therefore, it is not surprising that the MCU current density in Drosophila flight muscle is about four times lower than that in mouse heart. However, some mitoplasts originating from Drosophila tissues other than flight muscle have very high MCU current density, even exceeding the maximal MCU current density found in mice. Thus, in Drosophila , as seen in mice, MCU activity varies dramatically between tissues. Whether variations in MCU activity are due to tissue-specific regulation of the MCU (for example, via auxiliary subunits) or to different tissue-specific expression of the MCU channel requires further investigation. However, the tight control of MCU activity in highly active cells with intensive cytosolic Ca 2+ signalling is likely crucial for the normal physiology of these cells and for the integrity of their mitochondria. Misregulation of MCU activity in such tissues may lead to derangement of intracellular Ca 2+ signalling and mitochondrial dysfunction, followed by functional incompetence and degeneration. Isolation of mouse mitoplasts for patch-clamp recordings Mitoplasts were prepared from heart, skeletal muscle, liver, kidney and brown fat of adult (3–6-week-old) mice. Mitoplasts were isolated from wild-type C56BL/6 mice, except for brown fat mitoplasts obtained from mice deficient for uncoupling protein 1 (UCP1 −/−, C56BL/6 background, courtesy of Dr. Leslie Kozak, Pennington Biomedical Research Center, Louisiana State University, Baton Rouge, Louisiana, USA). Mice were killed by CO 2 asphyxiation followed by cervical dislocation. The selected mouse tissue was isolated, rinsed and homogenized in ice-cold medium containing 250 mM sucrose, 10 mM HEPES, and 1 mM EGTA (pH adjusted to 7.25 with KOH), using a glass grinder with six slow strokes of a Teflon pestle rotating at 280 (soft tissues) or 600 (fibrous tissues) rotations per minute. The homogenate was centrifuged at 700 g for 5–10 min to pellet nuclei and unbroken cells. For some tissues, the first nuclear pellet was resuspended in the same solution and homogenized again to increase the yield of mitochondria. Mitochondria were collected by centrifugation of the supernatant at 8,500 g for 10 min. Mitoplasts were produced from mitochondria using a French press. Briefly, mitochondria were suspended in a solution containing 140 mM sucrose, 440 mM D -mannitol, 5 mM HEPES, and 1 mM EGTA (pH adjusted to 7.2 with KOH), and then subjected to a French press at 2,000 psi to rupture the outer membrane. Mitoplasts were pelleted at 10,500 g for 15 min and resuspended for storage in 500 μl of solution containing 750 mM KCl, 100 mM HEPES and 1 mM EGTA (pH adjusted to 7.2 with KOH). Mitochondria and mitoplasts were prepared at 0–4 °C and stored on ice for up to 5 h. The French press method allows for a more gentle mechanical isolation of mitoplasts, and the pressure applied can be controlled to preserve the cristae of mitoplasts [29] . Immediately before the electrophysiological experiments, 15–50 μl of the mitoplast suspension was added to 500 μl of a solution containing 150 mM KCl, 10 mM HEPES and 1 mM EGTA (pH adjusted to 7.2 with KOH), and plated on 5-mm coverslips. For whole-mitoplast experiments, coverslips were pretreated with 0.1% gelatin to reduce adhesion. Only mitoplasts that had a figure 8-shaped appearance were selected for experiments, as this indicated the integrity of the matrix and membranes ( Fig. 1 ). Isolation of Drosophila mitoplasts The upstream activating sequence-MitoGFP [47] , [48] and Mef2-Gal4 (refs 47 , 49 ) flies were used as previously described. Flies were raised at 25 °C, and adult flies >5 days of age after eclosion were used. Drosophila mitoplasts were obtained from either the combined thoraces (devoid of legs and wings) of 70 flies or 30–50 whole-bodies of the Mef2 >MitoGFP flies. After grinding thoraces/whole flies with a Politron homogenizer for 3 min (rheostat set at 4), mitoplasts were obtained with the same protocol used for mouse mitoplasts (see above). Note that French-pressed Drosophila mitoplasts maintained the same figure 8-shaped morphology as seen in mouse mitoplasts (compare Figs 7a and 1 inset, white arrows). Patch-clamp recordings Mouse or Drosophila mitoplasts (2–6 μm in size) were used for patch-clamp experiments and typically had membrane capacitances of 0.3–1.3 pF. Currents were recorded using an Axopatch 200B amplifier (Molecular Devices). The voltage protocols and recording conditions are as indicated in the figures. Mitoplasts were stimulated every 5 s. To minimize errors in the voltage clamp associated with the liquid junction potential, a 3-M KCl-agar salt bridge was used as the bath reference electrode. Gigaohm seals with mitoplasts were formed in the bath solution containing 150 mM KCl, 10 mM HEPES and 1 mM EGTA, pH 7.2 (adjusted with KOH). Capacitative transients were completely compensated right after the seal was formed. Voltage steps of 350–500 mV from 15–50 ms were applied to rupture the IMM and obtain the whole-mitoplast configuration, as monitored by the appearance of capacitance transients and an increase in baseline noise. The access resistance and membrane capacitance of mitoplasts were determined using the Membrane Test tool of pClamp 10 (Molecular Devices). Typically, pipettes had resistances of 30–50 MΩ, and the access resistance was 40–80 MΩ. The averaged membrane capacitance of mitoplasts used in our experiments varied between tissues and was (0.65±0.04 pF, n =40) for skeletal muscle, (0.68±0.04 pF, n =13) for brown fat, (0.54±0.02 pF, n =18) for kidney, (0.36±0.02 pF, n =19) for liver, (0.67±0.02 pF, n =55) for heart and (1.31±0.06 pF, n =54) for Drosophila flight muscle. The calculated voltage clamp errors associated with the access resistance never exceeded 10 mV. Current amplitudes for histograms were measured within 5 ms after stepping the membrane from 0 to −160 mV. To measure Ca 2+ currents through the MCU, Figs 1 , 2 , 3 , 5 and 6 , pipettes were filled with 150 mM tetramethylammonium hydroxide, 1.5 mM EGTA, 1 mM MgCl 2 (2 mM MgCl 2 for Drosophila ), and 150 mM HEPES, pH 7.0 with D -gluconic acid, tonicity 450 mmol per kg (~330 mmol per kg for Drosophila ) with sucrose. In some experiments for Drosophila recordings, the tetramethylammonium hydroxide pipette solution was replaced with 110 mM Na-gluconate, 40 mM HEPES, 1.5 mM EGTA and 2 mM NaCl (pH adjusted to 7.0 with NaOH, tonicity adjusted to ~330 mmol per kg with sucrose). Whole-mitoplast control currents in Figs 1 , 2 , 3a , 5 , were recorded in a bath solution (HEPES/Tris solution) containing 150 mM HEPES and 1 mM EGTA (pH adjusted to 7.0 with Tris-base, tonicity adjusted to ~300 mmol per kg with sucrose). To record whole-mitoplast I MCU Ca 2+ currents ( Figs 1 , 2 , 3 , 5 and 6 ), a 1-M CaCl 2 stock solution was diluted to the final desired concentration in the HEPES/Tris solution without EGTA. To block I MCU Ca 2+ currents, RuR was added to the 100-μM Ca 2+ bath solution at a final concentration of 50 nM ( Fig. 7a ) or to the 1–5 mM Ca 2+ bath solution at a final concentration of 200 nM (left and right panels of Fig. 7b ). Bath solutions containing 100 μM–1 mM Ba 2+ or Mg 2+ were obtained by the addition of a 1-M stock solution of the corresponding chloride salt into the HEPES-Tris solution without EGTA. To study the monovalent current carried by MCU in DVF conditions ( Fig. 5 ), the following pipette solution was used: 110 mM Na-gluconate, 40 mM HEPES, 1 mM EGTA, 5 mM EDTA and 2 mM NaCl (pH adjusted to 7.0 with NaOH, tonicity adjusted to ~450 mmol per kg with sucrose). Bath solution used for these experiments contained: 110 mM Na-gluconate, 40 mM HEPES, 1 mM EGTA and 5 mM EDTA (pH 7.0 with NaOH, tonicity adjusted to 300 mmol per kg with sucrose). CaCl 2 was added to the Na-gluconate bath solution in the amount calculated by the MaxChelator winMaxC v2.05 programme (C. Patton, Stanford University) to obtain various free concentrations of Ca 2+ in the nanomolar range ( Fig. 4a ). For experiments in which we studied the permeability of the MCU to K + in the DVF conditions ( Fig. 4c ), the following bath solution was employed: 110 mM K-gluconate, 40 mM HEPES, 1 mM EGTA and 5 mM EDTA (pH 7.0 with KOH, tonicity adjusted to 300 mmol per kg with sucrose). All electrophysiological experiments were performed under continuous perfusion of the bath solution. Data acquisition and analyses were performed using PClamp 10 (Molecular Devices) and Origin 7.5 (OriginLab). All electrophysiological data presented were acquired at 10 kHz and filtered at 1 kHz. Statistical data are presented as the mean±s.e. All general chemicals as were purchased from Sigma (USA). How to cite this article: Fieni, F. et al . Activity of the Mitochondrial Calcium Uniporter Varies Greatly between Tissues. Nat. Commun. 3:1317 doi: 10.1038/ncomms2325 (2012).